Cavity cooling of free silicon nanoparticles in high vacuum Laser cooling has given a boost to atomic physics throughout the last 30 years, as it allows one to prepare atoms in motional states, which can only be described by quantum mechanics. Most methods rely, however, on a near-resonant and cyclic coupling between laser light and well-defined internal states, which has remained a challenge for mesoscopic particles. An external cavity may compensate for the lack of internal cycling transitions in dielectric objects and it may provide assistance in the cooling of their centre-of-mass state. Here we demonstrate cavity cooling of the transverse kinetic energy of silicon nanoparticles freely propagating in high vacuum (<10 −8 mbar). We create and launch them with longitudinal velocities down to v ≤1 m s −1 using laser-induced ablation of a pristine silicon wafer. Their interaction with the light of a high-finesse infrared cavity reduces their transverse kinetic energy by up to a factor of 30. Pioneering achievements in Doppler cooling [1] , [2] , polarization gradient cooling [3] or sub-recoil laser cooling [4] , [5] of atoms, and also the recently demonstrated Doppler cooling of molecules [6] , have opened rapidly growing fields of research in atomic and molecular physics. The accessibility of ultralow temperatures allows one to study even novel states of quantum degenerate matter [7] . In contrast to that, laser cooling of macromolecules or nanoparticles has been precluded by the lack of suitably narrow, closed optical transitions, which could be used to exchange momentum between light and matter. Off-resonant laser fields in high-finesse cavities may, however, be used to circumvent this restriction. Nanoparticles can then be cooled by applying an effective Sisyphus process, which forces them to climb in a sinusoidal optical potential, which is always higher in the ascent than in the descent. In practice, the potential hill arises from the dipole interaction between the particle’s polarizability and the electric field of the cavity’s standing light wave. Its amplitude is modulated by the particle itself when it crosses the nodes and antinodes of the cavity mode, and therefore changes the coupling of the field to the refractive index of the polarizable particle. The original idea of cavity cooling [8] , [9] has already been realized with atoms [10] , ions [11] and atomic ensembles [12] , even to below the recoil limit [13] . Such experiments benefit from advanced preparation methods and resonant optical forces, which are available for atoms. In contrast to that, the manipulation of mesoscopic particles cannot profit from any internal resonance. On the other hand, non-resonant light forces are non-satiating in nature and one can benefit from high optical intensities for cooling and from high scattering rates to gain detailed insight into the cavity-cooling process. Several groups have started to load silica (SiO 2 ) micro- or nanoparticles into buffer gas-assisted optical dipole traps to successfully subject them to optical cooling [14] , [15] , [16] . In contrast to that, we here demonstrate efficient transverse cavity cooling of pure and freely propagating silicon (Si) nanoparticles in a high-vacuum environment. Optical setup The outline of our experiment is shown in Fig. 1 . We generate pure silicon nanoparticles in situ by directing a pulsed focused laser beam onto the back side of a clean silicon wafer. The particles emerging from the front side travel upwards against gravity and interact with the standing light wave inside the high-finesse cavity. A fibre laser operating at λ =1,560 nm seeds the fundamental TEM 00 cavity mode. Its frequency is modulated via the double-pass acousto-optic modulator AOM1 and the locking signal is derived from the cavity mirror’s birefringence [17] . A part of the modulated laser light is split off, frequency modulated by 40 MHz in AOM2 and mixed with the light that is transmitted through the resonator on photodiode D3. The resulting 40 MHz beating signal is digitized to extract the phase difference between the two beams. 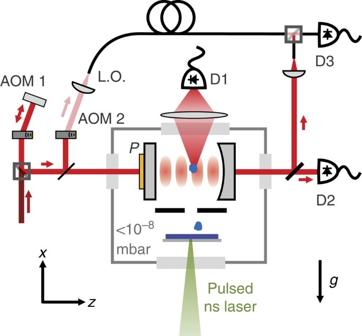Figure 1: Experimental setup for cavity cooling in a high-vacuum environment. The fibre laser beam (1,560 nm) is double passed in AOM1 (2 × 40 MHz) to stabilize the laser frequency to the cavity on short timescales. Over long timescales, the piezoelectric transducerPlocks the cavity to the laser frequency. A part of the stabilized beam is split off and frequency-shifted by AOM2 to serve as the local oscillator beam (LO). The other part (1 mW) is coupled into the high-finesse cavity inside a high-vacuum chamber (<10−8mbar). The cavity has a finesse of 3 × 105, a waist ofw=65 μm at the centre and consists of one flat and one curved mirror (radius of curvature: 25 mm). The transmitted intensity, which is a direct measure for the intracavity power, is detected by photodiode D2. A part of the transmitted intensity is fibre coupled, overlapped with the local oscillator beam and detected by D3. The phase of the resulting beating signal allows us to extract information about the cavity phase. A pulsed ns-laser (532 nm, 15 mJ) is focused onto a 0.5 mm thick silicon wafer to create and launch slow silicon nanoparticles. The wafer is attached to the top of a quartz plate. To avoid contamination of the cavity mirrors, the particles travel through a 1-mm aperture before they enter the cavity mode. Light scattered from within the cavity is focused onto the photodiode D1. Figure 1: Experimental setup for cavity cooling in a high-vacuum environment. The fibre laser beam (1,560 nm) is double passed in AOM1 (2 × 40 MHz) to stabilize the laser frequency to the cavity on short timescales. Over long timescales, the piezoelectric transducer P locks the cavity to the laser frequency. A part of the stabilized beam is split off and frequency-shifted by AOM2 to serve as the local oscillator beam (LO). The other part (1 mW) is coupled into the high-finesse cavity inside a high-vacuum chamber (<10 −8 mbar). The cavity has a finesse of 3 × 10 5 , a waist of w =65 μm at the centre and consists of one flat and one curved mirror (radius of curvature: 25 mm). The transmitted intensity, which is a direct measure for the intracavity power, is detected by photodiode D2. A part of the transmitted intensity is fibre coupled, overlapped with the local oscillator beam and detected by D3. The phase of the resulting beating signal allows us to extract information about the cavity phase. A pulsed ns-laser (532 nm, 15 mJ) is focused onto a 0.5 mm thick silicon wafer to create and launch slow silicon nanoparticles. The wafer is attached to the top of a quartz plate. To avoid contamination of the cavity mirrors, the particles travel through a 1-mm aperture before they enter the cavity mode. Light scattered from within the cavity is focused onto the photodiode D1. Full size image In parallel, the time evolution of the intracavity power is monitored via the intensity captured by D2 behind the cavity mirror R2. The photodiode D1, positioned under right angle to both the cavity axis and the polarization of the incident laser beam, is used to record the scattered light when a silicon particle passes the cavity. The detector is dominantly sensitive to the dipole radiation pattern, which reveals details about the coupling strength between the transiting particle and the cavity field. Cooling principle A subwavelength object of polarizability α experiences the optical potential V opt =− ħU 0 | a | 2 f 2 ( x ), where f ( x ) describes the intracavity mode function and a is the field amplitude. The particle effectively increases the cavity length due to its index of refraction and it shifts the cavity resonance by U 0 f 2 ( x ), where U 0 = αω L /2 ∈ 0 V , V is the mode volume and ω L is the angular frequency of the laser [18] . Because of the cavity’s high finesse, even a small length change leads to a significant phase shift of the cavity field. If the incident laser beam of frequency ω L is red-shifted with respect to the cavity resonance ω C ( ω L − ω C <0) any normal-dispersive particle (high-field seeker, index of refraction n >1) will tune the cavity resonance closer to the laser frequency and increase the intracavity power. When a particle moves along the cavity mode, it creates a time-dependent phase shift and intensity modulation. The intensity is maximal when the particle leaves an antinode of the optical lattice and is minimal when it moves towards it. Therefore, the particle gains less energy when it runs downhill than it loses while running uphill. This Sisyphus-type cooling [8] is most efficient when the field maxima coincide with the steepest slope of the coupling curve, which is satisfied for particles with a Doppler shift of | kv |≈|Δ|. To achieve the maximum intensity change per phase change, the cavity is detuned by one resonator line width κ to Δ ≈− κ . Particle launch One of the grand questions in nanoparticle cavity cooling, in comparison with the case of atoms, is how to prepare slow neutral particles in the first place. We use laser-induced thermo-mechanical stress on a pristine surface to generate and release clean silicon nanoparticles under high-vacuum conditions. The scanning electron micrograph (SEM) image in Fig. 2a shows a prototypical nanoparticle that was released from the front side of a silicon wafer when its back side was irradiated by pulsed laser light. This method generates objects of varying diameters and shapes, ranging from spheres of <100 nm across to arbitrarily shaped fragments well beyond 1 μm. An SEM image of the wafer’s front surface ( Fig. 2b ) corroborates the proposed mechanism of particle formation: microscopic cracks appear as a result of the laser-induced stress [19] . Here we post select the smaller fraction of particles, as objects with a radius above 200 nm will average over the standing wave potential and see reduced cooling forces [20] . 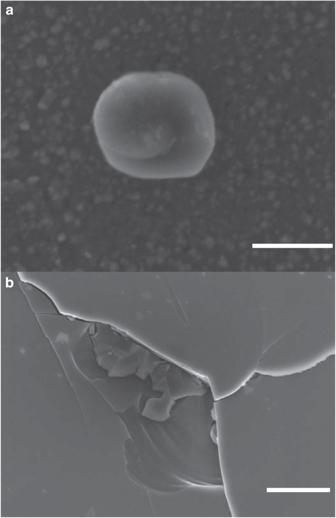Figure 2: Nanoparticle generation and launch. (a) An SEM image shows a typical silicon nanoparticle that is released by laser-induced thermo-mechanical stress ablation from a pure silicon (111) surface. Particles in the size range from below 100 nm to beyond 1,000 nm have been observed, with a variation of shapes. Although a full model of the release mechanism is still subject to future research, the cracks and defects on the front side of the back-irradiated silicon wafer (b) corroborate the hypothesis that micro cracks are the emission sites of nanosilicon. Energy-dispersive X-ray spectroscopy on the ejected nanomaterial allows us to identify silicon as the principal element, with oxygen as an occasional contaminant in some particles. Scale bar in (a) is 300 nm and in (b) is 1,000 nm. Figure 2: Nanoparticle generation and launch. ( a ) An SEM image shows a typical silicon nanoparticle that is released by laser-induced thermo-mechanical stress ablation from a pure silicon (111) surface. Particles in the size range from below 100 nm to beyond 1,000 nm have been observed, with a variation of shapes. Although a full model of the release mechanism is still subject to future research, the cracks and defects on the front side of the back-irradiated silicon wafer ( b ) corroborate the hypothesis that micro cracks are the emission sites of nanosilicon. Energy-dispersive X-ray spectroscopy on the ejected nanomaterial allows us to identify silicon as the principal element, with oxygen as an occasional contaminant in some particles. Scale bar in ( a ) is 300 nm and in ( b ) is 1,000 nm. Full size image Particle dynamics and cooling The light in photodiode D2 measures the intracavity power I c ( t ) and, therefore, also the expected optical forces. The intensity I s ( x ( t )) scattered into photodiode D1 is a measure for the light intensity at the particle position. We derive a normalized scattering coefficient S N ( t )≡( I s / I c )/max( I s / I c ) and plot it in Fig. 3a . It is an intensity-independent measure for the scattering probability, which contains information about the cooling process. It relates to the cavity mode function via S N ( t )=sin 2 ( kz ( t ))exp(−2 x 2 ( t )/ w 2 ), where w is the mode waist. We can extract the particle position z ( t ) from S N ( t ). When the particle passes the cavity with the velocity v x , we expect a Gaussian envelope of S N ( t ) with an e −1/2 half-width of w / v x . From this, we deduce an x velocity of v x =0.7 m s −1 for Fig. 3a . 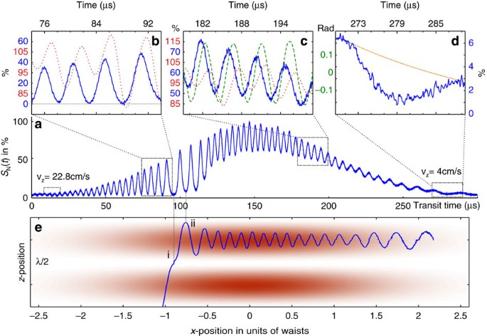Figure 3: Cavity cooling of a nanoparticle. (a) Cooling of a silicon nanoparticle traced by its scattered light in transit through the high-finesse infrared cavity. We plot the normalized scatteringSN(t) as a function of the particle’s transit time through the cavity mode. This allows us to extract the particle’s entrance and exit velocity along the cavity axis (d) and the particle trajectory (e). The modulation in the Gaussian envelope (b) is more pronounced in the entry wing than in the exit wing. This temporal asymmetry is indicative of cavity cooling, which reduces the velocity along the axis from 22.8(1) to 4.0(2) cm s−1. (b) When the particle enters the cavity mode, it runs over the standing wave and creates a sinusoidal modulation inSN(t) with 100% visibility (blue line). However, the cavity intensity (red dotted line) is modulated by the particle, although delayed because of the finite cavity response time. The intensity maxima coincide with the turning points ofSN(t), which corresponds to optimal cooling. (c) The particle is trapped and oscillates around the antinode. The cavity phase (green, dashed) is modulated by the particle with a slight time delay and the intensity (red, dotted) is again time delayed. Although the particle is trapped, it is still further cooled, as the intensity is still close to the maximal slope ofSN(t). When the particle leaves the centre of the Gaussian mode, the trapping frequency decreases again. (d) The evaluation of the particle transit time through the last oscillation in the exit wing ofSN(t) allows us to quantify the cavity cooling by comparing it with one of the first wiggles in the entrance wing. (e) Qualitative reconstruction of the particle’s trajectory in two spatial dimensions (see alsoSupplementary Fig. S5). The last free transit through a node of the standing light wave (i) and the first onset of trapping by the optical potential (ii) are correlated with the normalized scatteringSN(t) ofaat the times that are indicated by the dotted lines. Figure 3: Cavity cooling of a nanoparticle. ( a ) Cooling of a silicon nanoparticle traced by its scattered light in transit through the high-finesse infrared cavity. We plot the normalized scattering S N ( t ) as a function of the particle’s transit time through the cavity mode. This allows us to extract the particle’s entrance and exit velocity along the cavity axis ( d ) and the particle trajectory ( e ). The modulation in the Gaussian envelope ( b ) is more pronounced in the entry wing than in the exit wing. This temporal asymmetry is indicative of cavity cooling, which reduces the velocity along the axis from 22.8(1) to 4.0(2) cm s −1 . ( b ) When the particle enters the cavity mode, it runs over the standing wave and creates a sinusoidal modulation in S N ( t ) with 100% visibility (blue line). However, the cavity intensity (red dotted line) is modulated by the particle, although delayed because of the finite cavity response time. The intensity maxima coincide with the turning points of S N ( t ), which corresponds to optimal cooling. ( c ) The particle is trapped and oscillates around the antinode. The cavity phase (green, dashed) is modulated by the particle with a slight time delay and the intensity (red, dotted) is again time delayed. Although the particle is trapped, it is still further cooled, as the intensity is still close to the maximal slope of S N ( t ). When the particle leaves the centre of the Gaussian mode, the trapping frequency decreases again. ( d ) The evaluation of the particle transit time through the last oscillation in the exit wing of S N ( t ) allows us to quantify the cavity cooling by comparing it with one of the first wiggles in the entrance wing. ( e ) Qualitative reconstruction of the particle’s trajectory in two spatial dimensions (see also Supplementary Fig. S5 ). The last free transit through a node of the standing light wave (i) and the first onset of trapping by the optical potential (ii) are correlated with the normalized scattering S N ( t ) of a at the times that are indicated by the dotted lines. Full size image It is possible to reconstruct the particle trajectory with good reliability [21] to illustrate cooling and temporary channelling, as shown in Fig. 3 . In the beginning of the Gaussian envelope, the particle is almost unaffected by the weak optical potential and it travels under a small angle to the vertical direction. One expects a sinusoidal modulation of S N ( t ) with a period of T = λ /2 v z , where v z is the initial velocity along the cavity axis. A maximum in S N ( t ) reveals the particle’s passage through an antinode of the standing wave. When the nanosilicon approaches the cavity centre along the x axis, its transverse velocity v z is repeatedly reduced by the desired intracavity Sisyphus effect. Once the particle’s kinetic energy has fallen below the optical potential, the silicon ball is channelled vertically between two standing-wave nodes. The first velocity inversion, that is, the onset of channelling, can be identified with a first local non-zero minimum of S N ( t ). Near the first trapping point (i in Fig. 3e ), the oscillation period is particularly long, as the particle also explores the anharmonic part of the sinusoidal potential. On its way towards the centre of the Gaussian envelope, the particle experiences an increasing trap depth and it is further cooled. Therefore, the spatial excursions are then limited to the harmonic part of the well, resulting in faster oscillations. The oscillation amplitude of the channelled particle is a measure for its transverse kinetic energy and the cooling force is active as long as the intensity maximum lags behind the maximum of S N ( t ). However, the energy loss per cycle decreases, as the particle now remains bound to regions of similar coupling. The overall energy loss of the nanosilicon leads to a clearly visible asymmetry in S N ( t ). The particle enters the cavity with a horizontal velocity of v z =22.8(1) cm s −1 and leaves it with v z =4.0(2) cm s −1 . This corresponds to a reduction in the transverse kinetic energy by a factor of more than 30. While the particle moves along the standing-wave it modulates the cavity phase ( Fig. 3c ). From the amplitude of this modulation, we can extract an effective coupling frequency U z =2.3(4) κ . Because of an uncertainty in the y position, field averaging caused by the particle’s finite size and possibly an anisotropic shape, U z is a lower bound for the maximal coupling frequency U 0 . To estimate U 0 and to derive a particle size, we measure the trapping frequency f trap , while the particle is channelled. We find that the measured trapping frequency of f trap =145 kHz corresponds to a silicon sphere with a radius of about 150 nm (2 × 10 10 amu, polarizability of 4 π ∈ 0 × 2.7 × 10 9 Å 3 , N =7 × 10 8 atoms), which misses the cavity centre by about 0.4 waists. 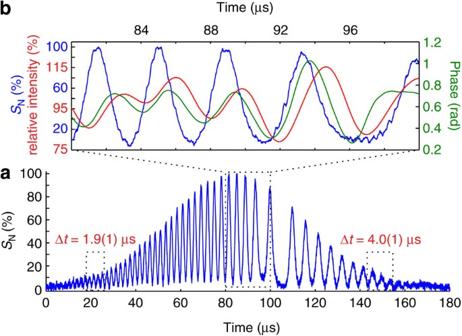Figure 4: Cavity cooling signals for a different nanosilicon particle. The particle’s initial and final transverse velocityvz,in=41(2) cm s−1andvz,out=20(1) cm s−1are derived from the modulation ofSN(a). The phase and intensity of the cavity respond with the time delay that is required for cooling (b). Figure 4a shows the normalized scattering signal S N ( t ) of a second nanoparticle in transit through the cavity. We find a forward velocity of v x =2.1 m s −1 . The initial transverse velocity is v z ,in =41(2) cm s −1 . Although the particle travels through the mode, the phase and intensity of the cavity lags behind S N , which leads to cooling (see Fig. 4b ). Contrary to the particle of Fig. 3 , this second particle runs over the standing wave, while leaving the cavity mode. Hence, the final transverse velocity can be measured directly as before and we obtain v z ,out =20(1) cm s −1 . The reduction of the transverse kinetic energy by a factor of 4.2(2) is smaller than for the particle in Fig. 3 . This can be explained by the higher forward velocity and the shorter interaction time with the cavity mode. Figure 4: Cavity cooling signals for a different nanosilicon particle. The particle’s initial and final transverse velocity v z ,in =41(2) cm s −1 and v z ,out =20(1) cm s −1 are derived from the modulation of S N ( a ). The phase and intensity of the cavity respond with the time delay that is required for cooling ( b ). Full size image The kinetic energy associated with the forward velocity is at least ten times larger than that related to the transverse component in our examples. Therefore, the forward velocity is less affected by the optical potential. In addition, electronic feedback suppresses intensity modulations on the timescale of the particle’s transit through the Gaussian waist but not during the particle’s passage between two cavity nodes. In summary, we do not expect a deviation from the overall Gaussian envelope. One may consider additional forces along the cavity axis different from the one mediated by the standing light wave. They are, however, estimated to be negligible in our case: an asymmetry of the dipole forces might be expected in z direction because of the asymmetric cavity configuration and the fact that the particles transit the field z =1.5 mm off-centre, that is, at half the cavity length. The z gradient of the laser field scales with the Rayleigh length as for z << z R =8 mm. Compared with the dipole forces that are related to the sinusoidal part of the cavity mode, this force asymmetry is smaller by a factor z / k =5 × 10 −6 . For highly transparent subwavelength particles, the net radiation pressure forces in a standing light wave field cancel [18] . The same number of photons arrives from both sides and the scattering events are balanced. For the same reason, we do not expect any asymmetric heating of the particle. Radiation pressure and dipole forces are also included in the general Mie calculation (see Methods). They become relevant for larger particles, as seen in Supplementary Fig. S1 . Photophoretic forces emerging from the interaction of a heated particle with its gaseous environment are completely negligible. At a residual pressure of P =10 −8 mbar, a 100-nm particle encounters a residual gas particle very rarely, on average every 300 μs. Moreover, a collision with a single N 2 or O 2 molecule will not impart any noticeable momentum kick onto the nanoparticle whose mass exceeds that of its collision partner by a factor 10 8 . We consider it a particular strength of our source design that we can exclude these environmental disturbances with certainty. Summarizing, we see substantial cavity cooling of pure silicon (Si) nanoparticles in a high-vacuum environment. The cavity-assisted readout also provides information about the particle’s polarizability, mass and velocity. Our demonstration is an important step towards quantum experiments with high mass particles. Although first new bounds on continuous spontaneous localization [22] , [23] will already come into reach with quantum interferometry at a mass range of 10 5 amu, certain tests will require nanoparticles of 10 8 –10 10 amu or more [24] . Objects that are big are, in principle, still compatible with an interferometer concept that prepares and probes quantum coherence using pulsed optical ionization gratings [25] , especially when working in the time domain (OTIMA) [23] . The work function of pure silicon (Si) is well matched to that. Future explorations of nonlinearities in quantum mechanics [22] , [26] , [27] , [28] , [29] will still require transit and coherence times of a few seconds at least. Our successful demonstration of cavity cooling by a factor of 30 in transverse energy is a promising starting point. It is interesting to consider multi-mode cavity cooling [30] to reduce the trapping forces close to the cavity centre to increase the cooling rate. Experiments are also on the way to extend the source to internally cold and mass-selected single particles on demand. Launching silicon nanoparticles in a high-vacuum environment Green light from a frequency-doubled Nd:YAG laser (Innolas, 532 nm, 15 mJ, 4 ns) is directed onto the back side of a 500-μm thick and chemically cleaned silicon wafer (111 cut), which is attached to a quartz plate and suspended in high vacuum (<1 × 10 −8 mbar). The origin of this method is similar to that of laser-induced acoustic desorption [31] , [32] with the difference that laser-induced acoustic desorption experiments are targeted at releasing surface adsorbents. Here we release nanomaterial from the pristine silicon surface itself by stress. The purity of the material is verified with energy-dispersive X-ray scattering inside an SEM. The particles are launched by the laser, but not necessarily in the same laser pulse that creates them. We also observe the formation of silicon dust on the front surface, which is then cleaned in subsequent laser shots. The fraction of observed particles that fall into the parameter range suitable for cooling amounts currently to ~1%. The parameter space is spanned by the size, lateral position and velocity of the particles. Most particles are still too big. They average over the standing wave and scatter so much that they may even extinguish the intracavity power. For that reason, they are also detected most easily. Silicon nanoparticles offer promising properties for cavity cooling as well as for future quantum interference studies alike. They exhibit a very high polarizability-to-mass ratio in comparison with many other dielectrics and are therefore well susceptible to optomechanical forces. Their high refractive index, n (1,560 nm)=3.47(1), is associated with a relative permittivity of ∈ = n 2 =12.04(1). Using the Clausus–Mosotti relation, we can relate the atomic polarizability and bulk permittivity, and find a value of α =4 πε 0 R 3 ( ∈ −1)/( ∈ +2). The work function of silicon is W =4.52 eV and indicates that single-photon ionization can easily be implemented using an ultraviolet or vacuum ultraviolet laser, as required for future OTIMA interference experiments [23] , [25] . Laser-cavity stabilization We use a fibre laser at 1,560 nm. It has a short-term (50 ms) line width of 20 kHz. Laser and cavity are locked by a slow and a fast feedback loop. Fast feedback is implemented via frequency modulation of the incident laser light in the double-pass AOM 1 ( Fig. 1 ). It operates with unity gain at 150 kHz. A slow active detuning and feedback loop is implemented by a piezoelectric displacement of the flat cavity mirror R1. This loop has a bandwidth of about 10 kHz. We exploit the intrinsic mirror birefringence to generate a dispersive locking signal without the need for actively modulating any optical element [17] . The high-finesse cavity is not only sensitive to the transiting nanoparticles but also to the tiny thermal expansion caused by the residual absorption in the mirror coating [33] , [34] . A rise in the intracavity intensity will lead to an even increased heating of the mirror coating and further thermal expansion. When the laser is red-detuned with respect to the optical cavity, this can result in self-stabilization but also in self-driven length oscillations with frequencies of the order of a few kilohertz in case of high laser intensities. To avoid these instabilities, the feedback modulation of the laser frequency must be fast enough. This fast feedback suppresses the slow cavity phase shift that is related to the particle’s passage through the Gaussian envelope along x . Only the oscillatory coupling along z remains, which is caused by the particle’s motion across the intracavity standing light wave. Time evolution of the cavity field The time evolution of the cavity field amplitude a ( t ) can be written as where η is the pump field, Δ is the laser-cavity detuning, κ is the cavity loss rate (line width), U 0 is the cavity shift and f ( x ) is the cavity mode function, which is explored by the particle moving along x ( t ). A formal integration of the cavity equation from time t =−∞ yields In the absence of any particle, the cavity assumes the stationary state a 0 = η /( κ − i Δ). To lowest order, a slowly moving particle would lead to a quasi-stationary field amplitude a ( t )≈ η /( κ − i (Δ+ U 0 f 2 ( x ( t )))). The formal solution (equation 2) describes the delayed reaction of the cavity to the moving sphere, which primarily modulates the phase of the field. As the cavity reaction timescale 1/ κ is finite, the particle-induced phase shift turns into an intensity modulation only after another delay. This explains the hierarchy of the observed phenomena in the cavity. The scattered light is an immediate signature of the particle position, followed by the delayed phase reaction of the cavity, and its intensity change, which reacts the slowest. Optical forces on a dielectric particle in a cavity mode The optical properties of the silicon particle in the presence of a linearly polarized standing-wave cavity field E 0 can be described using Mie-scattering theory [35] , [36] . The internal and scattering field components, E int and E sca , can be expressed in terms of a spherical wave expansion. The light-induced force acting on the sphere is then computed by integrating the Maxwellian stress tensor that is associated with the modified external field components E ext = E 0 + E sca and B ext over the sphere surface [37] . Apart from weak transverse forces due to the Gaussian profile of the cavity field, we find that the force F = F z e z is oriented along the standing-wave axis. We may express it in terms of the coupling frequency U z as F z =− ħkU z | a | 2 sin(2 kz )exp(−2( y 2 + x 2 )/ w 2 ). Supplementary Fig. S1 shows the transverse force for a point-like particle (green) compared with a full description (blue), which takes the finite particle size into account. For a sphere radius over R =120 nm, the force along the standing wave starts to deviate from the point particle approximation with the effective coupling frequency At a particle radius of about 190 nm, the force vanishes and it changes its sign for even larger radii. The force F z determines the motion along z [38] , where we assume that the particle traverses the cavity mode along the x axis. From this, we extract the harmonic frequency f trap for a particle trapped (channelled) at an antinode of the standing wave using , where P in is the incoupled power, and k =2 π / λ and c are the speed of light. We measure a frequency of 138 kHz at a normalized scattering S N =0.9 where the oscillation amplitude explores 33% of the trap potential. Taking the anharmonicity [39] into account, we deduce a harmonic trap frequency f trap =145 kHz. For a silicon point particle maximally coupled to the cavity mode, one expects f trap =183 kHz. The difference is attributed to the non-maximal coupling of a finite-sized particle. We measure U z =2.3(4) κ , which corresponds to the passage of a silicon sphere with a radius of ~150 nm that misses the cavity centre by 0.4 beam waists w y along the y axis. Velocity of the particle in the optical potential Because of cavity cooling, the velocity of the particle along z is reduced to a level at which it is influenced by even a small field in the exit wing of the Gaussian cavity beam. The corrugated optical potential modulates the velocity of the particle. At a maximum of the coupling, for instance, it is higher than outside the cavity mode. Assuming a static field amplitude and a constant velocity along x , the moving particle experiences the time-dependent force One can formally integrate the equation of motion to obtain For a weak potential, this can be approximated to first order by setting z ( t )= v 0 t , In Supplementary Fig. S2 , this expression (red) is plotted for a test particle together with its optical potential (blue). At an antinode/node of the field, the velocity is higher/lower than far out of the cavity mode. It oscillates around its final exit value v 0 . The particle velocity at finite coupling will be the same as far beyond the mode as long as the time spent at high and low potential averages out. To determine whether this is the case, we integrate the scattering intensity I S = I C S N ( t ) V opt ( t ) between the last two maxima over time, subtract the offset ( Supplementary Fig. S3 yellow area, A 1 ) and compare it with the area A 2 under the Gaussian envelope (area enclosed by the orange lines). If a particle spends more time at low fields, this will result in a smaller area under I S . For the numerical example of Supplementary Fig S2 , the ‘measured velocity’ v m at finite field and the ‘true final exit velocity’ v f at zero field will be equal and we find an area ratio of r A ≡2 A 1 / A 2 =1. In the parameter regime w / v x >> λ /2 v z , the Gaussian envelope causes only a negligible deviation of r A from 1. In contrast to that, a particle that is nearly or weakly trapped will spend more time in the low field region than in the high field. This results in r A <1 and the measured velocity v m would underestimate the true final velocity v f by the factor r v ≡ v m / v f <1. On the other hand, we obtain r v >1 if we overestimate the true velocity in our measurement. By simulating trajectories for different field strengths, we examine the correlation between r A and r v (see Supplementary Fig. S4 ). We distinguish two cases: particles that are trapped in the optical potential (blue dots) and untrapped particles travelling over the standing wave (red dots). For untrapped particles, the smaller the area ratio r A is, the more we underestimate the true velocity ( r v <1). For trapped particles (blue dots), we find r v <1 for r A ≲ 0.9 and r v >1 for 1> r A ≳ 0.9. Both the analytical and the numerical considerations show that the area ratio is a good measure for the validity of our method to extract the final velocity. For the particle studied in the main text ( Fig. 3 ), we obtain a ratio of r A =0.98(0.06), which assures that our measurement does not underestimate the true final exit velocity. Reconstruction of the particle trajectory We extract the particle position z ( t ) from the normalized scattering curve S N in the following manner. First, we divide S N by a fitted Gaussian envelope and then we take the inverse of the sinusoidal part. We assume the local maxima of S N to be positioned exactly at the antinodes of the standing light wave. We distinguish two sorts of local minima: those with a value near zero indicate that the particle passes through a node of the light field; non-zero minima appear at the reversal points, while the particle is channelled along an antinode of the standing wave. At both the maxima and the zero-valued minima, the coupling is insensitive to the particle’s change in position. This leads to discontinuities in the reconstruction of the trajectory, which are corrected with a linear regression. Supplementary Fig. S5 extends Fig. 3e in the main text by showing the full reconstruction from the particle’s entrance up to its exit of the Gaussian beam mode. Intensity noise-induced acceleration Successful cavity cooling requires that the local intensity maximum follows the maximum of the coupling curve in time, ideally with a phase lag of 90°. Only then the particle will climb higher than it falls in the potential well, which is modulated by the particle itself. This is clearly visible in Fig. 3b,c and in Fig. 4b . The complementary intensity-coupling correlation (phase lead of 90°) results in heating. To study this effect, one might consider tuning the laser from below to above the cavity resonance, that is, from Δ=− κ →Δ =+κ . A realization of this idea is, however, prevented by the thermal expansion of the mirror coating, which reduces the cavity length as a function of the intracavity laser intensity, admitting more light to it if the laser is initially blue-detuned. This leads to an instability and thermal runaway. However, imperfections in the laser-cavity stabilization lead to residual fluctuations of the intracavity intensity, which are uncorrelated to the particle dynamics. The intensity noise can therefore lead to temporary heating when the intensity maxima precede the maxima of the coupling curve in time. 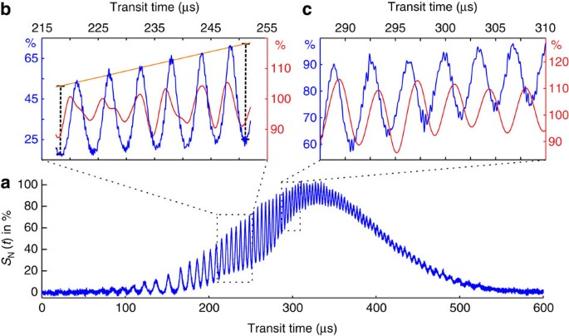Figure 5: Effect of intensity noise-induced heating. (a) Normalized scatteringSN(blue) of a third nanosilicon particle. (b) During a part of the trajectory, the intensity of the cavity fieldIc(red) incidentally fluctuates with a time delay toSNsuch that the particle is accelerated (heating). We extract the energy of the channelled particle by measuring the distance between the fitted Gaussian envelope (orange) and the turning points of the trapping oscillation (dashed black line). The energy results from the product of this difference and the cavity intensity (red curve). We find an increase of the transverse energy by ~14% over 40 μs. (c) Close to the centre of the Gaussian beam, the particle-induced intensity modulation dominates the intensity noise. Therefore, the particle is cooled. The overall cooling during the entire transit time by more than a factor of 8 is reflected in the asymmetry of the scattering curve (a). Figure 5 shows a particle traversing a blue-detuned cavity (adjusted for cooling as in Fig. 3 ). A comparison of the entrance and exit velocity shows again a net reduction of the transverse kinetic energy (that is, cooling). However, for the limited time span shown in Fig. 5b , the intracavity intensity noise increases the kinetic energy by ~14%. As expected for genuine cavity cooling/heating and as shown in Fig. 5c , this effect coincides with a phase slip (change of of sign) between the maxima of the intracavity intensity and the maxima of the coupling curve. Overall, the transverse kinetic energy of this third particle is reduced by more than a factor of 8. Figure 5: Effect of intensity noise-induced heating. ( a ) Normalized scattering S N (blue) of a third nanosilicon particle. ( b ) During a part of the trajectory, the intensity of the cavity field I c (red) incidentally fluctuates with a time delay to S N such that the particle is accelerated (heating). We extract the energy of the channelled particle by measuring the distance between the fitted Gaussian envelope (orange) and the turning points of the trapping oscillation (dashed black line). The energy results from the product of this difference and the cavity intensity (red curve). We find an increase of the transverse energy by ~14% over 40 μs. ( c ) Close to the centre of the Gaussian beam, the particle-induced intensity modulation dominates the intensity noise. Therefore, the particle is cooled. The overall cooling during the entire transit time by more than a factor of 8 is reflected in the asymmetry of the scattering curve ( a ). Full size image How to cite this article: Asenbaum, P. et al. Cavity cooling of free silicon nanoparticles in high vacuum. Nat. Commun. 4:2743 doi: 10.1038/ncomms3743 (2013).